Rapid control of phase growth by nanoparticles Effective control of phase growth under harsh conditions (such as high temperature, highly conductive liquids or high growth rate), where surfactants are unstable or ineffective, is still a long-standing challenge. Here we show a general approach for rapid control of diffusional growth through nanoparticle self-assembly on the fast-growing phase during cooling. After phase nucleation, the nanoparticles spontaneously assemble, within a few milliseconds, as a thin coating on the growing phase to block/limit diffusion, resulting in a uniformly dispersed phase orders of magnitude smaller than samples without nanoparticles. The effectiveness of this approach is demonstrated in both inorganic (immiscible alloy and eutectic alloy) and organic materials. Our approach overcomes the microstructure refinement limit set by the fast phase growth during cooling and breaks the inherent limitations of surfactants for growth control. Considering the growing availability of numerous types and sizes of nanoparticles, the nanoparticle-enabled growth control will find broad applications. Effective control of phase growth during material synthesis and processing is vital to achieve desired properties for materials [1] , [2] , [3] , [4] , [5] , [6] , [7] . Through decades of efforts, organic molecular and polymer surfactants are developed to control the size and morphology of phases for crystal growth and nanoparticle synthesis [4] , [8] . Recently, charged nanoparticles were used to control a slow crystal growth during gradual evaporation of aqueous solutions [9] . However, the low thermal stability and/or the sensitivity to chemical conditions prohibit their applications in numerous material systems during cooling under harsh conditions such as high temperature (which makes surfactant unstable and diffusion coefficient high), highly conductive liquids (which makes surfactant ineffective, for example, in metals and ionic liquids), dynamic chemical changes or high growth rate. Thus, the microstructure of these materials under harsh conditions is usually controlled by tuning growth time. However, for numerous materials with fast-growing speed, to obtain a fine microstructure, the growth time is normally controlled to be very short by using rapid cooling techniques, seriously limiting the sample size and processing window. Thus, novel approaches are needed to break these barriers for rapid control of phase growth under harsh conditions. Here we report a general method for rapid control of diffusional growth through effective physical growth restriction by rapidly self-assembling a layer of stable nanoparticles on the growing phase, which results in a uniformly dispersed phase orders of magnitude smaller than the one without nanoparticles. The effectiveness of this method is demonstrated in both inorganic and organic material systems for the growth control of liquid and solid phases at both low and high temperatures. Approach and model system The approach we developed for effective diffusional growth control is schematically shown in Fig. 1 . After phase nucleation, nanoparticles rapidly assemble on the growing phase to block diffusional transport ( Fig. 1a ), driven by a reduction in system interfacial energy ( Fig. 1b ). Since the adsorption of nanoparticles to the interface generally results in a reduction of interfacial area (indicated by solid blue line in Fig. 1b ), the suitable nanoparticles with a wide range of wetting angles to the growing and matrix phases will stay at the interface (see Supplementary Note 1 on the stability of nanoparticles at the interfaces and Supplementary Note 2 on nanoparticle selection criteria) with a much better stability than conventional surfactants under harsh conditions (see Supplementary Note 3 ). If a homogeneous nanoparticle is not available for a specific system, a Janus nanoparticle [10] (with one part likes the growing phase, while the other part likes the matrix) can be designed to ensure stability and thus effectively control its growth. 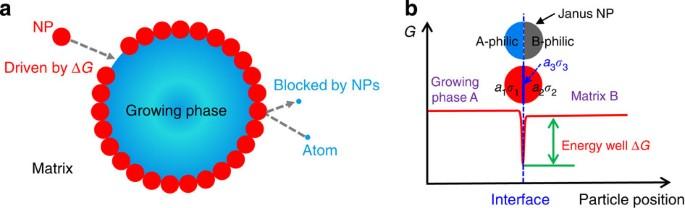Figure 1: Schematic illustration of phase growth control by nanoparticles. (a) The dispersed nanoparticles in matrix adsorb on the growing interface to block the diffusional transport of atoms to physically restrict the phase growth. (b) The nanoparticles assembly at the growing interface is driven by a reduction in system interfacial energy.a1as NP/growing phase interfacial area,a2as NP/matrix interfacial area,a3as the lost growing phase/matrix interfacial area because of the presence of NP, andσ1,σ2,σ3are NP/growing phase, NP/matrix, growing phase/matrix interfacial free energies, respectively. The reduction in interfacial areaa3(free energy ofa3σ3) always drives nanoparticles to the growing phase/matrix interface. In case thata3σ3is not large enough to stabilize nanoparticles on the growing interface, in principle, for any growing interface, a Janus nanoparticle (with one part likes the growing phase, while the other part likes the matrix) can be designed to stay firmly at the growing interface for growth control. Figure 1: Schematic illustration of phase growth control by nanoparticles. ( a ) The dispersed nanoparticles in matrix adsorb on the growing interface to block the diffusional transport of atoms to physically restrict the phase growth. ( b ) The nanoparticles assembly at the growing interface is driven by a reduction in system interfacial energy. a 1 as NP/growing phase interfacial area, a 2 as NP/matrix interfacial area, a 3 as the lost growing phase/matrix interfacial area because of the presence of NP, and σ 1 , σ 2 , σ 3 are NP/growing phase, NP/matrix, growing phase/matrix interfacial free energies, respectively. The reduction in interfacial area a 3 (free energy of a 3 σ 3 ) always drives nanoparticles to the growing phase/matrix interface. In case that a 3 σ 3 is not large enough to stabilize nanoparticles on the growing interface, in principle, for any growing interface, a Janus nanoparticle (with one part likes the growing phase, while the other part likes the matrix) can be designed to stay firmly at the growing interface for growth control. Full size image The effectiveness of this approach is verified in both inorganic and organic material systems for the growth control of liquid and solid phases at both low and high temperatures. Immiscible alloy, well known for its exceptionally fast growth of phases and extremely harsh conditions (for example, high temperature, high conductivity and high growth rate) during cooling/solidification, was selected as a model system to elucidate the scientific principle of nanoparticle-enabled growth control in detail. We will demonstrate and discuss the effectiveness of this method in other material systems (for example, eutectic alloy and organic materials) later. Immiscible alloys are alloys with a miscibility gap in the liquid state, having a wide range of potential applications [5] , [6] , [11] , [12] , [13] , [14] , [15] , [16] . However, immiscible alloys proved extremely difficult to process [5] , [6] , [7] , as illustrated with a typical immiscible alloy Al–Bi [17] in Fig. 2 . As seen in its phase diagram ( Fig. 2a ) [18] , above the miscibility gap the alloy components are completely miscible as a single solution. When this homogenous liquid is cooled down into the miscibility gap, a new liquid phase with distinct properties nucleates. The diffusion coefficient in liquid alloys is generally very high (up to 10 −8 m 2 s −1 , 10 orders of magnitude higher than the one in solid, typical of 10 −18 m 2 s −1 ) [5] ; therefore once nucleated, the minority liquid droplets can grow very rapidly to become large droplets, which are prone to coalescence and segregations [5] , [7] , [19] , as illustrated in Fig. 2b . A rapid cooling rate of at least hundreds of Kelvin per second is usually needed to reduce the time for diffusional growth of the minority liquid phases. Unfortunately, the high temperature gradient under the rapid cooling generally induces severe thermocapillary forces [7] , [19] that push the droplets to the hotter region. This dilemma makes the uniform dispersion of the fine minority droplets have not been achieved in immiscible alloys by regular casting for the past 100 years. 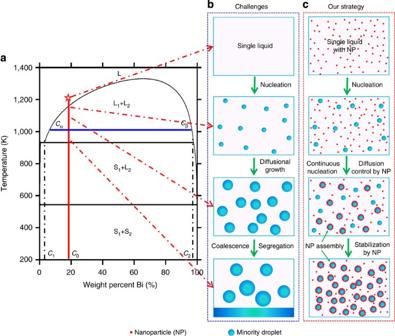Figure 2: Challenge and our strategy for fast-growing phase control. (a) Phase diagram of a typical immiscible alloy Al-Bi. (b) Schematic of the structure evolution during the cooling of an immiscible alloy. Above the miscibility gap, the alloy components are completely miscible as a single phase. During cooling, the minority phase liquid droplets nucleate and grow rapidly by diffusion, then coalesce and settle down to bottom under gravity and/or move to the center driven by thermocapillary force in a short time. (c) Our strategy for growth control of minority phase droplets by nanoparticles during cooling of immiscible materials. Nanoparticles are dispersed uniformly in the single solution above miscibility gap. During the cooling through the miscibility gap, they spontaneously assemble at the interface between the nucleated minority droplets and the liquid matrix, rapidly forming a dense, thin nanoparticle coating on the minority droplets to significantly block the diffusional transport to greatly limit their growth. The rapid and effective diffusional growth restriction by nanoparticles enables a continuous nucleation of new droplets during the whole period of cooling, because of effectively limiting the consumption of supersaturated solute by the droplets nucleated first and significant reduction of latent heat released. In addition, the thin nanoparticle coating will also effectively resist the coalescence by introducing a high capillary pressure in the liquid film between the approaching nanoparticle-coated droplets. Since the driving forces (gravity and thermocapillary) for segregation are not significant on very small droplets, a uniform distribution of very small droplets can be readily obtained. Figure 2: Challenge and our strategy for fast-growing phase control. ( a ) Phase diagram of a typical immiscible alloy Al-Bi. ( b ) Schematic of the structure evolution during the cooling of an immiscible alloy. Above the miscibility gap, the alloy components are completely miscible as a single phase. During cooling, the minority phase liquid droplets nucleate and grow rapidly by diffusion, then coalesce and settle down to bottom under gravity and/or move to the center driven by thermocapillary force in a short time. ( c ) Our strategy for growth control of minority phase droplets by nanoparticles during cooling of immiscible materials. Nanoparticles are dispersed uniformly in the single solution above miscibility gap. During the cooling through the miscibility gap, they spontaneously assemble at the interface between the nucleated minority droplets and the liquid matrix, rapidly forming a dense, thin nanoparticle coating on the minority droplets to significantly block the diffusional transport to greatly limit their growth. The rapid and effective diffusional growth restriction by nanoparticles enables a continuous nucleation of new droplets during the whole period of cooling, because of effectively limiting the consumption of supersaturated solute by the droplets nucleated first and significant reduction of latent heat released. In addition, the thin nanoparticle coating will also effectively resist the coalescence by introducing a high capillary pressure in the liquid film between the approaching nanoparticle-coated droplets. Since the driving forces (gravity and thermocapillary) for segregation are not significant on very small droplets, a uniform distribution of very small droplets can be readily obtained. Full size image To address this grand challenge, here we use our nanoparticle assembly approach to control the diffusional phase growth under cooling through rapidly coating the growing phase with thermally stable nanoparticles, as illustrated in Fig. 2c . When suitable nanoparticles are dispersed in the alloy solutions, during the cooling through the miscibility gap, they spontaneously assemble at the interface between the nucleated minority droplets and the liquid matrix, rapidly forming a dense, thin nanoparticle coating on the minority droplets to significantly retard, if not completely block, the diffusional transport to greatly limit their growth ( Fig. 2c ). The rapid and effective physical diffusion control of phase growth by nanoparticles can substantially block the growth of the early nucleated droplets and enable a continuous formation of new droplets during the whole period of cooling. In the system without nanoparticles, the nuclei can only form at the beginning of the phase separation. During cooling of the pure system, the fast growth of the droplets nucleated first will immediately consume the supersaturated solute in the surrounding melt and increase the temperature of the surrounding melt by releasing latent heat. Consequently, the surrounding melt does not have chance to form new nuclei even with effective inoculant particles because of a lack of sufficient undercooling/supersaturation. Thus, the total number of the nuclei is mostly limited to the number of the nuclei initially formed at the beginning of cooling in the pure system. In contrast, with the rapid and effective diffusional growth restriction by nanoparticles, the surrounding melt can gain sufficient undercooling/supersaturation for a continuous nucleation of new droplets during the whole period of cooling, due to effectively limiting the consumption of supersaturated solute by the droplets nucleated first and significant reduction of latent heat released. Thus, the total number of the nuclei formed in the system with nanoparticles are substantially higher than that without nanoparticles, which will result in a much finer microstructure. In addition, we took inspirations from the strategy of using molecular surfactants and solid particles to control the coalescence of emulsions [20] , [21] , [22] , [23] . The thin nanoparticle coating will also effectively resist the coalescence by introducing a high capillary pressure in the liquid film between the approaching nanoparticle-coated droplets. The effectiveness of this strategy is demonstrated in detail in Al-Bi alloy, one of the most difficult immiscible alloys to control the rapid phase growth [17] , by using TiC 0.7 N 0.3 nanoparticles (The selection of TiC 0.7 N 0.3 was guided by the nanoparticle selection criteria as shown in Supplementary Note 2 . Also see Methods, Supplementary Figs 1 and 2 ). 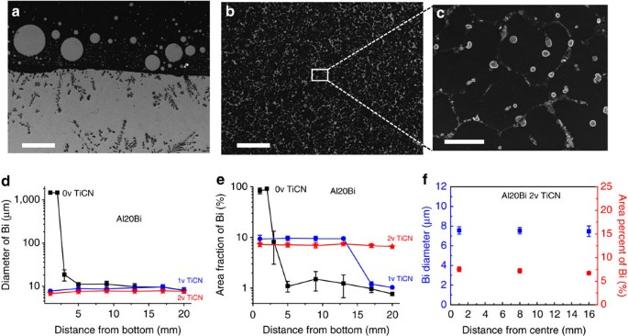Figure 3: Distribution of the minority Bi Phase. SEM images of the pure Al-20Bi alloy (a) and Al-20Bi alloy with 2 vol.% TiC0.7N0.3nanoparticles (b,c) cooled under a cooling rate of 1 K s−1. Bi diameter (d) and Bi area fraction (e) at different distances from the bottom. (f) Bi diameter and area fraction at different distances from the centre of Al-20Bi alloy with 2 vol.% TiC0.7N0.3nanoparticles. The Bi phase settles down to the bottom, forming a thick layer of Bi in pure alloy. Remarkably, with incorporation and dispersion of 2 vol.% TiC0.7N0.3nanoparticles into the melt, a uniform distribution of Bi phase with diameter in the micrometre range was obtained. Scale bars, 500 μm in (a,b), 50 μm in (c). Error bars represent s.d. of three data sets. The dispersion and size of the Bi phase Figure 3a shows the backscattered scanning electron microscopy (SEM) image taken from the bottom part of the solidified monolithic Al-20wt.% Bi (hereafter noted as Al-20Bi) alloy. As expected, the Bi phase settles down to the bottom, forming a thick layer of Bi with ~12 vol.% of the precipitated Al phase. The thickness of the Bi layer at the bottom is ~2.5 mm, accounting for about 90 vol.% of the total Bi in the sample. This confirms that the Bi in the monolithic Al-20Bi alloy segregates severely during solidification. Remarkably, when we used ultrasonic processing to disperse 2 vol.% TiC 0.7 N 0.3 nanoparticles into the Al-20Bi alloy, no sedimentation was observed ( Fig. 3b,c ) after a cool down under a low cooling rate of 1 K s −1 . We further analysed the distribution of Bi phase in the pure alloy and samples with 1 and 2 vol.% of TiC 0.7 N 0.3 nanoparticles versus the distance from the bottom of the samples, as shown in Fig. 3d for average diameters and Fig. 3e for area fractions, respectively. With the incorporation of only 1 vol.% of TiC 0.7 N 0.3 nanoparticles, the distribution of Bi is improved dramatically, while some minor sedimentation to the bottom region of the sample still exists. However, with 2 vol.% of TiC 0.7 N 0.3 nanoparticles, both the size and area fraction of Bi are very uniform throughout the sample. The average size of Bi droplets is ~7.5 μm. To check whether thermocapillary force induced non-uniformity, the distribution of Bi phase from the centre to the edge along the horizontal direction in the Al-20Bi alloy sample with 2 vol.% TiC 0.7 N 0.3 nanoparticles (hereafter noted as Al-20Bi-2vTiCN) was analysed. The results ( Fig. 3f ) show that the Bi phase is also distributed uniformly along the horizontal direction, indicating that thermocapillary force induced little pushing of Bi droplets to the centre. The uniform distribution of a high percentage of micrometre-sized Bi droplets is observed throughout the sample of the Al-20Bi-2vTiCN, even though it was produced under a very low cooling rate of 1 K s −1 . Figure 3: Distribution of the minority Bi Phase. SEM images of the pure Al-20Bi alloy ( a ) and Al-20Bi alloy with 2 vol.% TiC 0.7 N 0.3 nanoparticles ( b , c ) cooled under a cooling rate of 1 K s −1 . Bi diameter ( d ) and Bi area fraction ( e ) at different distances from the bottom. ( f ) Bi diameter and area fraction at different distances from the centre of Al-20Bi alloy with 2 vol.% TiC 0.7 N 0.3 nanoparticles. The Bi phase settles down to the bottom, forming a thick layer of Bi in pure alloy. Remarkably, with incorporation and dispersion of 2 vol.% TiC 0.7 N 0.3 nanoparticles into the melt, a uniform distribution of Bi phase with diameter in the micrometre range was obtained. Scale bars, 500 μm in ( a , b ), 50 μm in ( c ). Error bars represent s.d. of three data sets. Full size image The distribution of the TiC 0.7 N 0.3 nanoparticles We then investigated the distribution of the TiC 0.7 N 0.3 nanoparticles in the solidified samples with field emission SEM (FESEM) and transmission electron microscopy (TEM), and sought to verify the interfacial assembly of the nanoparticles. As shown in Fig. 4a–d , the nanoparticles form a thin layer coating (randomly and closely packed, but not fused together) on Bi droplet, which indicates that the TiC 0.7 N 0.3 nanoparticles prefer to stay at the interface between Bi and Al. 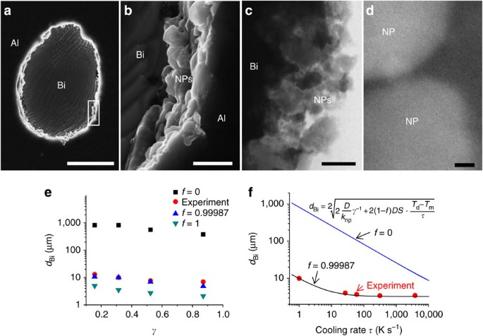Figure 4: TiC0.7N0.3nanoparticles (NPs) coating on the Bi phase and effective control of diffusional growth. (a) SEM image of a Bi droplet with nanoparticle coating. To see nanoparticle coating clearly, ion milling was used to preferentially remove Bi away to reveal the nanoparticle shell on the droplets of Bi. (b) Magnified view of the area in the box ina. The SEM images show that the nanoparticles form a dense coating on the surface of Bi droplets. (c) Bright field (BF) TEM image of nanoparticle coating on the surface of Bi phase. The nanoparticles are randomly and closely packed on the surface of Bi phase. (d) High-angle annular dark-field (HAADF) TEM image of two closely packed nanoparticles. A gap of ~1 nm is observed between two closely packed nanoparticles. (e) Bi size as a function of γ=Cnp/Sunder a cooling rate of 1 K s−1. Droplet sizes are plotted from experimental results and theoretical predictions with various diffusion blocking efficienciesf. (f) Bi size as a function of the cooling rate for Al-20Bi-2vTiCN. Without diffusional growth control (diffusion blocking efficiencyf=0), the size of the Bi phase is orders of magnitude larger than the experimental value. The small droplet size can only be obtained with high diffusion blocking efficiency (f=0.99987). Scale bars, 5 μm ina, 500 nm inb, 200 nm incand 5 nm ind. Figure 4: TiC 0.7 N 0.3 nanoparticles (NPs) coating on the Bi phase and effective control of diffusional growth. ( a ) SEM image of a Bi droplet with nanoparticle coating. To see nanoparticle coating clearly, ion milling was used to preferentially remove Bi away to reveal the nanoparticle shell on the droplets of Bi. ( b ) Magnified view of the area in the box in a . The SEM images show that the nanoparticles form a dense coating on the surface of Bi droplets. ( c ) Bright field (BF) TEM image of nanoparticle coating on the surface of Bi phase. The nanoparticles are randomly and closely packed on the surface of Bi phase. ( d ) High-angle annular dark-field (HAADF) TEM image of two closely packed nanoparticles. A gap of ~1 nm is observed between two closely packed nanoparticles. ( e ) Bi size as a function of γ =C np / S under a cooling rate of 1 K s −1 . Droplet sizes are plotted from experimental results and theoretical predictions with various diffusion blocking efficiencies f . ( f ) Bi size as a function of the cooling rate for Al-20Bi-2vTiCN. Without diffusional growth control (diffusion blocking efficiency f =0), the size of the Bi phase is orders of magnitude larger than the experimental value. The small droplet size can only be obtained with high diffusion blocking efficiency ( f =0.99987). Scale bars, 5 μm in a , 500 nm in b , 200 nm in c and 5 nm in d . Full size image Stability of nanoparticles at interface It is known that the stability of the solid nanoparticles assembled at the liquid–liquid interface is determined by the Brownian motion energy and the energy needed to remove the particles from the interface to the bulk liquid phases [24] . The latter is: where r is the radius of the particles, σ is the interfacial free energy between the two liquids, θ is the contact angle, measured through the liquid 1 on the solid particle in the environment of liquid 2, and the ‘+’ sign refers to particle removal into the bulk liquid 2 phase, while the ‘−’ sign refers to the removal of the particle into the bulk liquid 1 phase [24] . The Brownian motion energy ( E b ) is: where k is the Boltzmann constant (1.3806503 × 10 −23 m 2 kg s −2 K −1 ) and T is the absolute temperature of the liquids. In the system of Al-Bi alloy with TiC 0.7 N 0.3 particles, the average nanoparticle radius, r , is ~40 nm, interfacial free energy σ between Al and Bi liquid is ~16 mN m −1 at 1,173 K 11 and T is ~1,173 K. The wetting angle was experimentally estimated to be ~128° (see Fig. 5 ). Thus, the energy (Δ G ) needed to remove the nanoparticle from the interface to the bulk liquid phases is estimated to be ~1 × 10 −17 J, which is more than three orders of magnitude higher than the Brownian motion energy of the particles ( E b ), 8 × 10 −21 J, at 1,173 K ( Fig. 5 ). Therefore, a deep interfacial energy well effectively traps the TiC 0.7 N 0.3 nanoparticles at the interfacial region between the Bi and Al phases, as illustrated in Fig. 4b . 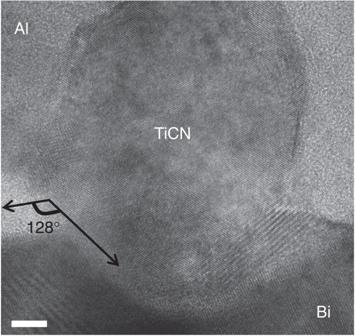Figure 5: Wetting angle. The wetting angle of 128° was estimated from the triple junction in the TEM image of TiC0.7N0.3nanoparticle at the Bi and Al interface for calculation of the energy needed to remove the particles to the bulk liquid phases. Scale bar, 5 nm. Figure 5: Wetting angle. The wetting angle of 128° was estimated from the triple junction in the TEM image of TiC 0.7 N 0.3 nanoparticle at the Bi and Al interface for calculation of the energy needed to remove the particles to the bulk liquid phases. Scale bar, 5 nm. Full size image Diffusional growth control We further investigated the diffusional growth of the Bi droplets with and without the nanoparticle coating. Assuming the Bi droplets nucleate and grow only by diffusional transport of Bi, the diameter of Bi can be determined by: where D is the diffusion coefficient, t is the cooling time in the immiscible region and S is the supersaturation, a temperature-dependent parameter [25] . The average S can be calculated by: where C 0 is the Bi concentration in the matrix, and C 1 and C 2 are the concentrations of the Al-rich and Bi-rich liquid at monotectic temperature, respectively (as shown in Fig. 2a ). The estimated average Bi droplet size through diffusional growth would be ~821 μm for pure Al-20Bi alloy following equation (3), which is two orders of magnitude larger than the experimental value of 7.5 μm for Al-20Bi-2vTiCN. This clearly indicates that without an effective control of diffusional growth it would be impossible to obtain micrometre-sized Bi droplets at a low cooling rate (about 1 K s −1 ) for pure Al-20Bi alloy. Thus, the nanoparticles must have greatly reduced the diffusional growth of the Bi droplets during cooling/solidification. We have constructed a theoretical model to better understand the remarkable diffusional growth control of Bi droplets by TiC 0.7 N 0.3 nanoparticles by assuming an irreversible adsorption model for nanoparticles to assemble on the surface of droplet (see Supplementary Note 4 and Supplementary Fig. 3 ). In this model, f is defined as the diffusion blocking efficiency by the nanoparticle coating, C np as the concentration of nanoparticles and t np as the characteristic time (time constant) for nanoparticle coverage on the droplets. t np is a function of the size, density and volume percentage of nanoparticles, nanoparticle stacking factor, nanoparticle adsorption efficiency and melt temperature. C np and t np can be related by a constant k np as: When t np << t, It should be noted that the equation (6) only considers diffusional growth before the monotectic temperature. The extremely small Bi droplets formed after the monotectic temperature were thus excluded, so that the experimental data can be compared more accurately with the theoretical one. We experimentally estimated k np and f by casting the Al-20Bi-2vTiCN melt to a copper wedge mold to cool the alloy melt at different cooling rates (see Supplementary Note 5 and Supplementary Table 1 ). The k np and f were determined, using equation (6), to be ~11,340 s −1 and 0.99987, respectively, from the measured droplet sizes obtained at different cooling rates. The t np for Al-20Bi-2vTiCN was estimated to be ~4.4 ms. The short t np shows that the nanoparticles can rapidly coat the droplets completely within a few milliseconds. The remarkable high diffusion blocking efficiency f confirms that the nanoparticle coating is effective to control diffusional growth. If we define γ=C np /S, the dependence of the Bi droplet size on γ was experimentally investigated by varying the volume percentages of nanoparticles ( C np ) and Bi concentration. Using the k np and f values experimentally determined from Al-20Bi-2vTiCN samples, we theoretically determined the Bi droplet size for the experimentally studied γ . The theoretical values match the experimental ones very well ( Fig. 4e ). To show the influence of the diffusion blocking efficiency on droplet sizes, we also calculated the Bi droplet diameter as a function of γ for the cases of f =0 (that is, no nanoparticles and no diffusional growth control) and f =1 (that is, assuming the nanoparticle coating totally blocked the diffusion; Fig. 4e ). The data clearly suggest that the nanoparticle-enabled diffusional growth control is the key to obtain the remarkably small Bi droplets in this work. Furthermore, Fig. 4f shows the dependence of the experimental and calculated Bi droplet diameters on cooling rates for Al-20Bi alloy. The cooling time was calculated by t =( T d − T m )/ τ , where T d and T m are the decomposition temperature and monotectic temperature, respectively, and τ is the cooling rate. Without diffusional control (that is, f =0), the droplet size is large and strongly depends on the cooling rate. However, with a nanoparticle-enabled diffusional barrier ( f =0.99987), the droplet size is not only orders of magnitude smaller but also depends little on cooling rates, especially when the cooling rate is higher than 50 K s −1 (corresponding to an approximate cooling time t =10 3 t np ). The average Bi sizes depend on the competition between t np and (1− f ) t . With a remarkable high diffusion blocking efficiency of f =0.99987 in this study, at a cooling rate that yields a cooling time of about 40 s (~6 K s −1 in Al-20Bi), t np starts to dictate the Bi particle size, effectively eliminating the need for high cooling rates demanded by conventional processing methods. The model developed here elucidates the fundamental principle of diffusional growth control by nanoparticle coating. On the basis of the theoretical analysis, the criteria for nanoparticle selection were summarized for a rational design of new materials (see Supplementary Note 2 ). The nanoparticles at the droplet interface are also effective for suppressing coalescence [24] , [26] . Figs. 6a,b show that the TiC 0.7 N 0.3 nanoparticles trapped at the surface of Bi droplets can stabilize the Bi droplets against coalescence when two Bi droplets collide with each other induced by hydrodynamic motions. The SEM image and energy-dispersive X-ray spectroscopy (EDS) analysis of the boundary region between the two small Bi droplets ( Fig. 6b,d ) further validate that a thin layer of nanoparticle-stabilized Al separates the two Bi droplets against coalescence. Interestingly, some submicrometre-sized Bi droplets, located along the Al grain boundary, were also stabilized by nanoparticle coatings ( Supplementary Fig. 4 ). Past studies showed that solid particles could stabilize the thin liquid film between two approaching droplets by increasing the pressure needed to break the thin liquid film [24] , [26] , as schematically shown in Fig. 6c . Using parameters for the Al-Bi-TiC 0.7 N 0.3 nanoparticle system, the pressure is estimated to be 3.48 MPa in the liquid Al film between the approaching Bi droplets ( Supplementary Note 6 ). Such high pressure can effectively resist coalescence. 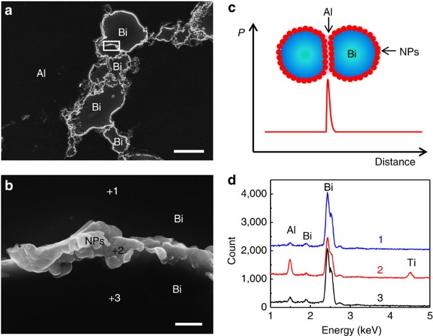Figure 6: TiC0.7N0.3NPs coating for effective control of coalescence. (a) SEM image of a Bi droplet cluster. (b) Magnified view of the area in the box ina. (c) Schematic of the capillary pressure in the liquid film between two colliding nanoparticle-coated droplets. The nanoparticles raise the pressure to break the thin liquid film between two colliding droplets to against coalescence. (d) EDS of the interface region between two Bi droplets. The high intensity of the Ti and Al peaks indicates that two Bi droplets are separated by TiC0.7N0.3NP stabilized Al thin film. Scale bars, 10 μm inaand 500 nm inb. Figure 6: TiC 0.7 N 0.3 NPs coating for effective control of coalescence. ( a ) SEM image of a Bi droplet cluster. ( b ) Magnified view of the area in the box in a . ( c ) Schematic of the capillary pressure in the liquid film between two colliding nanoparticle-coated droplets. The nanoparticles raise the pressure to break the thin liquid film between two colliding droplets to against coalescence. ( d ) EDS of the interface region between two Bi droplets. The high intensity of the Ti and Al peaks indicates that two Bi droplets are separated by TiC 0.7 N 0.3 NP stabilized Al thin film. Scale bars, 10 μm in a and 500 nm in b . Full size image The properties of the materials (cut from the middle part of the ingots) were evaluated by friction and tensile tests ( Supplementary Fig. 5 and Supplementary Note 7 ). The Al-20Bi-2vTiCN exhibits a remarkably lower, by one order of magnitude, coefficient of friction (COF). The significant reduction in COF indicates that our approach is very effective and has immediate practical application for development of high performance bearing alloys with ultralow COF to substantially reduce the energy loss of numerous engines. In principle, the concept of our approach can be used to control the growth of any phases by adsorption of nanoparticles to the phase interfaces. We selected methanol (CH 3 OH)-cyclohexane (C 6 H 12 ), which is a system used for chemistry education [27] , to demonstrate the application of our nanoparticle approach for growth control in organic system. In this system, the Ostwald ripening rate is very high because of the high mutual solubility of methanol and cyclohexane. When the sample is kept at two-liquid region at room temperature before observation, Ostwald ripening will result in the growth of the larger droplets at the expense of the smaller ones [28] . In addition to controlling the supersaturation-driven diffusional growth during cooling, the nanoparticle coating will also effectively control the Ostwald ripening [29] , [30] . We identified the nanoparticle (B 4 C) for growth control in this system according to our nanoparticle selection criteria ( Supplementary Note 2 ). With the growth control by nanoparticles, more than one order of magnitude reduction in droplet size is achieved as compared with the pure system ( Fig. 7a–c and Supplementary Note 8 ). We also demonstrate that our approach is effective to control the growth of solid phase by nanoparticles in a eutectic alloy, Al-Sn system ( Fig. 7d–f and Supplementary Note 9 ). 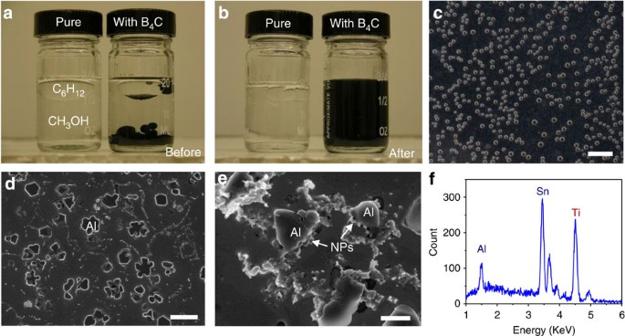Figure 7: Growth control by nanoparticles in organic system and for solid–liquid interface. (a–c) Fifty-nanometre boron carbide (B4C) nanoparticles control the growth of C6H12in CH3OH-40 vol.% C6H12system during cooling. (a) At room temperature, ~15 vol.% C6H12is immiscible with CH3OH in this system, segregating to top of the vial (outer diameter of 34 mm). When B4C nanoparticles (black powder) are poured into the liquid from top, some nanoparticles are trapped at the liquid–liquid interface, some particles even form a complete coating on the surface of the C6H12droplets (which were created during nanoparticle pouring). This clearly shows that B4C nanoparticles prefer to stay at the CH3OH–C6H12interface. (b) After heating up the solution to the single phase region and dispersing B4C nanoparticle uniformly in the single phase liquid by ultrasonic processing, the liquids were cooled down from single solution region to room temperature without ultrasonic radiation. With B4C nanoparticles, a uniform emulsion is obtained, while in pure sample the C6H12forms big droplets and segregates to top of the vial. (c) Optical microscopy image shows that the C6H12droplets are uniform with a diameter of ~20 μm, which is more than one order of magnitude smaller than the calculated droplet size in pure sample (assuming the droplet only grows by diffusion). (d–f) TiC0.7N0.3nanoparticles control the growth of Al phase in Sn-6.8wt.%Al alloy. (d) SEM image shows that primary Al phase grows to large dendrite structure in pure Sn-6.8Al during solidification. (e) However, the size of the Al phase in Sn-6.8Al+2 vol.% TiC0.7N0.3nanoparticle sample is much smaller than the size of the Al phase in pure Sn-6.8Al; the nanoparticle coating on the surface of the primary Al phase was clearly observed by in-lens detector. (f) EDS spectrum of the particles ineindicates that the nanoparticles are TiC0.7N0.3. Scale bars, 100 μm inc, 20 μm indand 2 μm ine. Figure 7: Growth control by nanoparticles in organic system and for solid–liquid interface. ( a – c ) Fifty-nanometre boron carbide (B 4 C) nanoparticles control the growth of C 6 H 12 in CH 3 OH-40 vol.% C 6 H 12 system during cooling. ( a ) At room temperature, ~15 vol.% C 6 H 12 is immiscible with CH 3 OH in this system, segregating to top of the vial (outer diameter of 34 mm). When B 4 C nanoparticles (black powder) are poured into the liquid from top, some nanoparticles are trapped at the liquid–liquid interface, some particles even form a complete coating on the surface of the C 6 H 12 droplets (which were created during nanoparticle pouring). This clearly shows that B 4 C nanoparticles prefer to stay at the CH 3 OH–C 6 H 12 interface. ( b ) After heating up the solution to the single phase region and dispersing B 4 C nanoparticle uniformly in the single phase liquid by ultrasonic processing, the liquids were cooled down from single solution region to room temperature without ultrasonic radiation. With B 4 C nanoparticles, a uniform emulsion is obtained, while in pure sample the C 6 H 12 forms big droplets and segregates to top of the vial. ( c ) Optical microscopy image shows that the C 6 H 12 droplets are uniform with a diameter of ~20 μm, which is more than one order of magnitude smaller than the calculated droplet size in pure sample (assuming the droplet only grows by diffusion). ( d – f ) TiC 0.7 N 0.3 nanoparticles control the growth of Al phase in Sn-6.8wt.%Al alloy. ( d ) SEM image shows that primary Al phase grows to large dendrite structure in pure Sn-6.8Al during solidification. ( e ) However, the size of the Al phase in Sn-6.8Al+2 vol.% TiC 0.7 N 0.3 nanoparticle sample is much smaller than the size of the Al phase in pure Sn-6.8Al; the nanoparticle coating on the surface of the primary Al phase was clearly observed by in-lens detector. ( f ) EDS spectrum of the particles in e indicates that the nanoparticles are TiC 0.7 N 0.3 . Scale bars, 100 μm in c , 20 μm in d and 2 μm in e . Full size image Our approach reported here is fundamentally different from growth control by surfactants and breaks the inherent limitations of surfactants (see Supplementary Note 3 ). Our approach is also conceptually different from earlier work on inoculation in melt solidification and overcomes the microstructure refinement limit set by the fast phase growth during melt solidification (see Supplementary Notes 10 and 11 , and Supplementary Figs. 6 and 7 ). Since numerous types and sizes of nanoparticles will be available, the nanoparticle-enabled growth control will have a tremendous impact by effectively controlling the growth of phases in numerous systems. This nanoparticle approach would also enable broad and practical processing windows for production of numerous materials through solution methods. The nanoparticle-enabled mechanism for a rapid and effective control of diffusional transport would be of interests for diverse fields such as materials science, chemistry, biology and physics (see Supplementary Note 12 ). Melt preparation and nanoparticle dispersion Al-Bi melt was prepared by melting commercial pure aluminium (99.5%, AA1350) and bismuth (99.9%, Alfa Aesar) in an alumina crucible using an electrical resistance furnace. TiC 0.7 N 0.3 nanoparticles (shown in Supplementary Fig. 1 , with an average diameter of ~80 nm, from Sigma-Aldrich) were fed and dispersed into the molten metal by an ultrasonic cavitation-based method (schematically shown in Supplementary Fig. 2 ) [31] . Supplementary Fig. 2b illustrates the schematic of the experimental setup for the melt preparation and ultrasonic processing. The resistance heating furnace was used to heat Al-Bi melt to designed temperature in an alumina crucible with a diameter of 36 mm. The inert gas protection system was used to protect the melt and nanoparticles from oxidation by injecting argon through two nozzles. The nanoparticle-feeding system was used to feed nanoparticles into the melt. In this study, a double-capsulate feeding method was used. Nanoparticles were wrapped with 0.0127-mm-thin Al foil (alloy 1000), and then the Al foil was rolled into a rod shape with a diameter of ~6 mm (making the first capsule). The Al foil rod, containing the nanoparticles, was wrapped again with another thin Al foil (alloy 1100) with a dimension of 355.6 × 152.4 × 0.0254, mm (making the second capsule). The second Al foil would make the nanoparticles discharge into the melt gradually, resulting from a gradual melting of the thicker wall of the capsule. The ultrasonic processing system consists of an ultrasonic probe, booster and transducer. An ultrasonic probe made of niobium alloy C103 with a diameter of 12.7 mm and a length of 175 mm was attached to a booster (Sonicator 3000, Misonix Inc), which was mounted in a transducer working under a frequency of 20 kHz and a maximum 600-W power output. When the Al-Bi alloy was melted in the alumina crucible at 973 K, the tip of the niobium ultrasonic probe was inserted ~6 mm in depth into the melt. Ultrasonic vibration with a frequency of 20 kHz and a peak-to-peak amplitude of 60 μm was generated from the transducer. Then the preheated nanoparticles (at 423 K for 1 h) were added into the melt with the double-capsulate feeding method during ultrasonic processing. Each double capsulate can carry ~1 vol.% of nanoparticles into the melt. It took 15 min to disperse the nanoparticles released from one capsulate by the ultrasonic processing. After feeding and dispersing nanoparticles at 973 K, the ultrasonic probe was lifted out of the melt. Then the melt was heated to 1,183 K (above the miscibility gap for this composition). To make sure nanoparticles are well dispersed before cooling, the melt was treated again by ultrasonic processing for 15 min at 1,183 K. Solidification and cooling rate measurement After ultrasonic processing, the ultrasonic probe was lifted out of the melt. For low cooling rate experiments, the crucible was taken out of the furnace. The Al-Bi melt with nanoparticles was cooled down inside the crucible in air (as shown in Supplementary Fig. 2 ). For comparison, the pure Al-Bi alloy was also prepared under the same conditions (except no nanoparticles). We measured the cooling rate by inserting thermocouples inside the melt during cooling. The cooling rate before solidification is ~1 K s −1 . For high cooling rate experiments, the melt was cast to a copper wedge mold to cool the alloy melt at different cooling rates. The cooling rate was calculated using an empirical equation from the thickness of the sample [32] . Structure characterization After solidification, the distribution of the minority Bi phase was studied with FESEM (Zeiss LEO 1530) using backscattering electron imaging. The area fraction and average size of the Bi phase were calculated from the backscattering images using the software ImageJ. The nanoparticle distribution and bonding with the matrix were investigated with FESEM and high-resolution TEM (HRTEM, FEI Titan 80–200 Aberration-corrected (S)TEM). Owing to a preferential etching of Bi by both electropolishing and ion milling, the samples for HRTEM were cut by focused ion beam mill (FIB, Zeiss 1540 XB CrossBeam Workstation) to reduce the preferential etching. Sample preparation procedure for nanoparticle distribution study In order to understand how the TiC 0.7 N 0.3 nanoparticles stabilize the Bi phase, we investigated the interfacial assembly of the TiC 0.7 N 0.3 nanoparticles in the solidified samples with FESEM. First we tried to observe the TiC 0.7 N 0.3 nanoparticle distribution from the sample prepared by traditional metallurgical polishing. Approximately 30 s before the end of polishing, alcohol was poured on the polishing cloth to rinse the sample. Then the sample was cleaned by sonication. Even though we cleaned the sample so carefully, some nano-sized polishing powders still stick on the surface, seriously interfering with the TiC 0.7 N 0.3 nanoparticles under SEM observation. To solve the problem, the sample was cleaned by low angle ion milling for 2 h with milling parameters of 4 kV voltage, 4 mA current, 15° milling angle and 360° stage rocking angle. After ion milling, only embedded TiC 0.7 N 0.3 nanoparticles remain on the sample, which was confirmed with electron EDS. Wetting angle determination It is difficult to determine the wetting angle of TiC 0.7 N 0.3 nanoparticles with Bi in the environment of Al [33] . Here we cut a TEM sample from the boundary between Bi and Al by FIB and observed the triple junction formed by TiC 0.7 N 0.3 nanoparticle, Bi and Al with HRTEM. The wetting angle of TiC 0.7 N 0.3 nanoparticles with Bi in the environment of Al before a completed solidification can be estimated from the geometry of the triple junction, as shown in Fig. 5 . Property characterization The samples for testing were cut from the middle part of the solidified Al-20Bi and Al-20Bi-2vTiCN ingots. Coefficients of friction were tested by using Ball-on-Disk Tester (D9.625-mm steel ball, 2-kg normal force) at 0.63 mm s −1 (slow) and 0.83 mm s −1 (fast) scratching speeds in air without any lubrication. The yield strength, tensile strength and tensile elongation were tested by uniaxial tensile testing (Shimazu AGS-20kNG, gauge length 10 mm, strain rate 1 × 10 −3 s −1 ). How to cite this article: Chen, L.-Y. et al. Rapid control of phase growth by nanoparticles. Nat. Commun. 5:3879 doi: 10.1038/ncomms4879 (2014).